Electroformation of Janus and patchy capsules Janus and patchy particles have designed heterogeneous surfaces that consist of two or several patches with different materials properties. These particles are emerging as building blocks for a new class of soft matter and functional materials. Here we introduce a route for forming heterogeneous capsules by producing highly ordered jammed colloidal shells of various shapes with domains of controlled size and composition. These structures combine the functionalities offered by Janus or patchy particles, and those given by permeable shells such as colloidosomes. The simple assembly route involves the synergetic action of electro-hydrodynamic flow and electro-coalescence. We demonstrate that the method is robust and straightforwardly extendable to production of multi-patchy capsules. This forms a starting point for producing patchy colloidosomes with domains of anisotropic chemical surface properties, permeability or mixed liquid–solid phase domains, which could be exploited to produce functional emulsions, light and hollow supra-colloidosome structures, or scaffolds. Janus and patchy particles whose surfaces are composed of two or more patches of different chemical or physical properties [1] , [2] , [3] , is a rapidly developing research topic [4] , [5] , [6] , [7] , [8] . A central vision is to design these particles such that they can self-assemble into simple or complex architectures [3] , [9] , [10] . Janus or patchy particles can be fabricated by various means [11] , [12] , [13] , [14] and, recently, several experimental realizations of their self-organization have been reported, which include self-assembly of colloidal patchy spheres into colloidal kagome lattices [15] , colloidal ‘molecules’ [16] and other structures [17] , [18] , [19] . Through this kind of ‘bottom-up’ process, two- or three-dimensional small clusters or larger entities can be produced, and these may serve as scaffolds suitable for biomedical applications [20] , in assembling electric circuits [21] or optical structures such as photonic crystals [22] , and as vehicles for liquid or molecular transport [23] . Janus and patchy capsules are distinct from Janus and patchy particles, and they combine functionalities, offered by Janus [1] , [2] or patchy [3] particles, and those given by capsules such as colloidosomes [24] , [25] . Hollow capsules with controlled permeability are promising candidates for functional encapsulation of entities such as molecules, particles or bubbles, and is becoming increasingly important for a wide variety of applications [26] . Homogenous colloidal shells or colloidosomes (made out of one type of material) are routinely made by precipitation polymerization, inverse suspension polymerization techniques, or typically by emulsion-based methods [25] , [27] . However, the formation of heterogeneous shells (made out of at least two types of material) is challenging. Here we show that both Janus and more advanced patchy capsules can be assembled by combining electro-coalescence and electro-hydrodynamic (EHD) flow in leaky dielectric [28] emulsion drops. The starting configuration of the method is two or several leaky dielectric drops embedded in another leaky dielectric fluid and already partly covered by colloidal or larger particles at chosen concentration. The particles are trapped in the liquid interface by capillary forces [29] . The particles can be brought to the drop interface by any suitable method of choice, such as EHD flow [30] , microfluidic methods [31] or simple mechanical stirring [32] . Recently [30] , it was demonstrated how EHDs induce self-organization of colloidal particles on such drop surfaces, that is, particles are transported by means of Taylor EHD flow into the drop ‘electric equator’. This enables electro-coalescence of the partly covered drops into highly ordered jammed colloidal shells with domains of controlled size and composition (in the following, shell refers to the wall of the capsule). We also demonstrate that the method is straightforwardly extendable to production of multi-patchy capsules, simply by subsequent electro-coalescence of several droplets in a row. This hydrodynamically based assembly route is robust, as it requires neither direct manipulation of the particles by the electric field, nor interaction between the particles themselves. This means that any type of insulating or weakly conductive particles can be used. Our novel assembly route involves the simultaneous action of EHD flow and electro-coalescence that is different from previously reported methods, such as layer-by-layer surface coating of colloidal particles followed by subsequent dissolution of the colloidal core [33] , [34] , and targeted hydrodynamic delivery of colloidal particles on drops by micro-fluidics flow devices [31] . Furthermore, the route allows for the final functional capsule to be made out of any type of insulating or weakly conductive materials. Behaviour of drops in E-fields We consider here a system of two immiscible leaky dielectric fluids where one of the fluids carries drops of the other fluid. The leaky dielectric drops experience both dielectrophoretic and electrohydrodynamic interactions [35] . For drops aligned in the electric field direction, the dipole interaction is always attractive, whereas the EHD interaction can be repulsive or attractive depending on the relative conductive and dielectric permittivity of the liquids. If the charge relaxation time of the drop is longer than that of the surrounding liquid, the drops attract [35] . The hydrodynamic attraction or repulsion is determined by the charge relaxation time, which determines the direction of the flow. As the relaxation time of castor oil and silicone oil is ~\n1 and 20 s, respectively, the EHD flow is attractive in the present case. The relative velocity of attracting drops strongly depends on the distance between drops. The EHD force is dominant at long distances and the dielectrophoretic force governs when drops are sufficiently close to one another [35] . EHD effects are not present in an AC field, as there is no free charge build-up on the drop interface, and in this case the system behaves like a perfect dielectric (rather than a leaky dielectric). We have observed that applied DC fields result in much faster coalescence than AC fields, suggesting that long-range EHD attraction is important for bringing the drops in contact. Formation of Janus capsules The right panel (experimental part) of Fig. 1 shows two silicone oil drops in castor oil. The drop surfaces are covered with polyethylene (PE) particles (with green and red fluorescent dyes) forming ribbon structures in an electric DC field. The volume of each drop is ~\n1.5 μl and the concentration of PE particles corresponds to 5% of the drop weight. Initially, the distance between the drop centres is around 4 R , where R is the radius of a drop, and the particles are distributed uniformly on the drop surfaces. An external DC electric field of 200 V mm −1 is applied (at t =0 s) in the horizontal direction. Ribbons are formed at the drop electric equators. Driven by the attractive EHD and electrostatic forces, the drops approach one another. In the experiment shown in Fig. 1 it takes ~\n145 s to reduce the separation distance from ~\n4 R to 2 R . At this point, there is still a thin film of castor oil separating the drops. An additional 40 s are required for this layer to thin out and the remaining film to rupture, allowing the drops to coalesce. Electro-coalescence of Pickering droplets can exhibit unusual dynamics due to breakup of coalescent bridges by the colloidal particles [36] . Here we do not observe this unusual coalescence dynamics because the coalescence region is particle-free. After coalescence occurs, a Janus shell is formed rapidly in a few seconds. The coalesced drop is now fully covered by particles. During the coalescence, the particles can move and reorganize only within the drop surfaces due to the strong desorption energies [29] . The close-up of the structure (right panel of Fig. 1 ) in the Janus shell shows that particles are closely packed and arranged in slightly disordered hexagons (see also Supplementary Fig. 1 ). Turning off the electric field does not induce any observable movement of the particles in the shell, that is, the shell is stable. However, if the coalesced drop is not fully covered by particles (for example, when particles form a ribbon), the particles may move on the drop surface and sediment when the electric field is turned off. 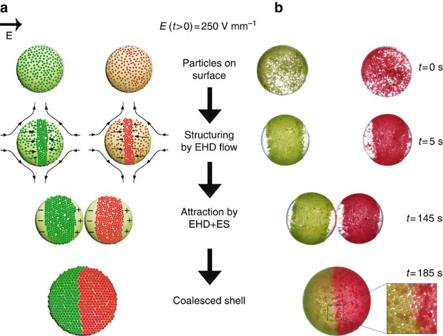Figure 1: The fabrication process. (a) The sketch of Janus capsule assembly and (b) images from an experiment. Before an external DC electric field is applied (t<0 s), particles occupy the surface of the drop at random. After the DC electric field is applied, the drop becomes a dipole. It takes only few seconds to bring particles away from the ‘electric poles’ of the drop to the drop ‘electric equator’ by EHD flow induced by a DC electric field (E=250 V mm−1in this experiment). The two drops with ribbon-like structures attract one another by both the EHD and electro static (ES) forces. Finally, the drops electro-coalesce, resulting in the formation of densely packed Janus shell. Turning off the electric field does not induce observable particle movement in the shell, that is, the shell is stable, as the particles are arranged in a jammed, slightly disordered hexagonal structure as shown in the blow-up. The electric field direction is horizontal in the plane of the panels. The size of the PE particles is 50±3 μm. Figure 1: The fabrication process. ( a ) The sketch of Janus capsule assembly and ( b ) images from an experiment. Before an external DC electric field is applied ( t <0 s), particles occupy the surface of the drop at random. After the DC electric field is applied, the drop becomes a dipole. It takes only few seconds to bring particles away from the ‘electric poles’ of the drop to the drop ‘electric equator’ by EHD flow induced by a DC electric field ( E =250 V mm −1 in this experiment). The two drops with ribbon-like structures attract one another by both the EHD and electro static (ES) forces. Finally, the drops electro-coalesce, resulting in the formation of densely packed Janus shell. Turning off the electric field does not induce observable particle movement in the shell, that is, the shell is stable, as the particles are arranged in a jammed, slightly disordered hexagonal structure as shown in the blow-up. The electric field direction is horizontal in the plane of the panels. The size of the PE particles is 50±3 μm. Full size image At the electric field strengths used in our experiments, saturated drops formed by coalescence do not subsequently coalesce with other drops. However, we cannot exclude the possibility that a saturated drop coalesce with another drop if higher electric fields strengths are used. In Fig. 2 and the corresponding Supplementary Movie 1 we show coalescence of two drops each with a thinner ribbon as compared with that presented in Fig. 1 . In this case there is clearly a visible EHD flow in the coalesced drop, as the two ribbons are brought together. The particles in Fig. 2 are located on the drop surface, before and after coalescence, which is also the case for covered drops, as shown in Supplementary Fig. 2 . 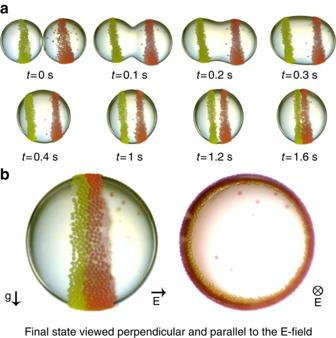Figure 2: Coalescence of drops with thin PE ribbons. (a) Dynamics of coalescence of drops with thin ribbons. (b) Final state viewed perpendicular and parallel to the electric field direction. After a rapid coalescence, the two ribbons are carried by EHD circulation flows. The electric field is horizontal, except in the lower right panel, which is a view of the final state parallel to the electric field, showing that the particles are located on the drop’s surface. See also the correspondingSupplementary Movie 1. The size of the coalesced drop is about 1.5 mm. The gravity is in the vertical direction as indicated by the arrow. Figure 2: Coalescence of drops with thin PE ribbons. ( a ) Dynamics of coalescence of drops with thin ribbons. ( b ) Final state viewed perpendicular and parallel to the electric field direction. After a rapid coalescence, the two ribbons are carried by EHD circulation flows. The electric field is horizontal, except in the lower right panel, which is a view of the final state parallel to the electric field, showing that the particles are located on the drop’s surface. See also the corresponding Supplementary Movie 1 . The size of the coalesced drop is about 1.5 mm. The gravity is in the vertical direction as indicated by the arrow. 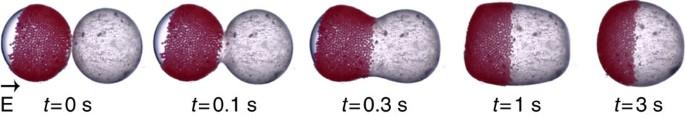Figure 3: Amphiphilic Janus colloidal capsules. Coalescence of a Janus colloidal capsule made of hydrophobic red PE particles and hydrophilic fluorohectorite clay particles. The clay particles on the right hemisphere of the shell are completely packed, they are individually not visible and the shell appears translucent. The coalescence is fast and the dynamics depend on the viscosity of the dispersed phase. See also the correspondingSupplementary Movie 2, which shows the drop coalescence and how fast the shell is made. The clay and the PE particles form a stable interface, indicating that both the clay and the PE particles are jammed. The size of the coalesced drop is about 1.5 mm. Full size image Figure 3 demonstrates that the method also works for a wider range of particles. The images in Fig. 3 show coalescence of two drops covered by red PE particles and synthetic clay colloidal particles. The resulting Janus colloidal capsule comprises two materials with different electrical properties, sizes, porosity and wettability. Clay particles are hydrophilic and the PE particles are hydrophobic, that is, an amphiphilic shell is formed. The clay particles on the right hemisphere of the shell are completely packed, and so small that the shell appears translucent. Supplementary Movie 2 shows the drop coalescence and how fast the shell is made. We note that the clay particles, which can be as small as 5 μm or less, do not diffuse into the 50-μm PE layer. Figure 3: Amphiphilic Janus colloidal capsules. Coalescence of a Janus colloidal capsule made of hydrophobic red PE particles and hydrophilic fluorohectorite clay particles. The clay particles on the right hemisphere of the shell are completely packed, they are individually not visible and the shell appears translucent. The coalescence is fast and the dynamics depend on the viscosity of the dispersed phase. See also the corresponding Supplementary Movie 2 , which shows the drop coalescence and how fast the shell is made. The clay and the PE particles form a stable interface, indicating that both the clay and the PE particles are jammed. The size of the coalesced drop is about 1.5 mm. Full size image In the present assembly approach, it is possible to use insulating or weakly conductive particles with dielectric properties similar to that of the host fluid, such as polymers, glass, or mineral particles such as clays. Particles with higher conductivity, such as metal particles, cannot be used in this approach as they form conducting dipolar chains that repel one another and suppress the essential electrohydrodynamic flows [30] . It has previously been shown that stable shells can be made from particles with sizes as small as 100 nm (ref. 37 ). The lower size limit is generally determined by the particle–interface binding energy, which decreases significantly with particle size, and may become comparable with Brownian thermal energies. 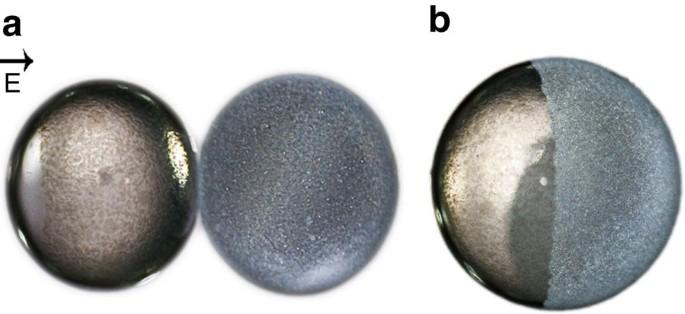Figure 4: Janus colloidal capsule. (a) Two drops with ribbon-like structures assembled from PS and glass particles just before coalescence. (b) The drops electro-coalesced, resulting in the formation of a densely packed Janus colloidal capsule. The size of the coalesced drop is ~\n1.5 mm and the size of the colloidal particles is 500 and 1,000 nm, left and right hemisphere, respectively. Figure 4 shows a Janus colloidal capsule comprising monodisperse glass particles of sizes 500 and 1,000 nm, respectively. We have also looked at smaller drop sizes, as demonstrated in Supplementary Fig. 3 , where 1 μm particles formed a ribbon on a ~\n50-μm diameter coalesced droplet. Figure 4: Janus colloidal capsule. ( a ) Two drops with ribbon-like structures assembled from PS and glass particles just before coalescence. ( b ) The drops electro-coalesced, resulting in the formation of a densely packed Janus colloidal capsule. The size of the coalesced drop is ~\n1.5 mm and the size of the colloidal particles is 500 and 1,000 nm, left and right hemisphere, respectively. Full size image Non-spherical capsules The coalescence of two drops of the same size reduces the available surface area by ~\n20%, leading to a more densely packed particle layer than in the two original drops. If the original particle concentration on the two original drops is sufficiently high, the coalescence can lead to ‘arrested coalescence’ [37] where the particles form a rigid film that resists the Laplace pressure gradient, which attempts to drive the coalesced drop towards a spherical shape. Four examples of such arrested capsules are shown in Fig. 5 . 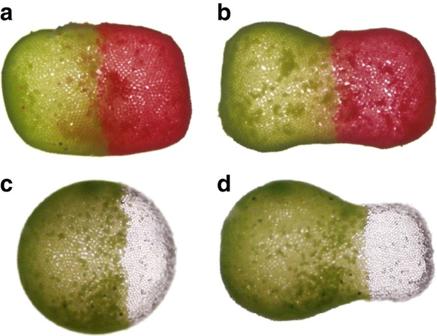Figure 5: Asymmetric Janus capsules after turning off the electric field. (a,b) Coalesced drops with equal material proportion. PE (50 μm green and red) particle concentration 7 wt% (a) and 10 wt% (b). The drops are non-spherical and remain so throughout the course of the experiment. (c,d) Coalesced drops with tuned material proportion. The original drops had different volumes (2:1 ratio) before coalescence. (c) Spherical capsule made of drops with 5 wt% particles, PE (green) and PS (white). (d) The bulb-like capsule was achieved by increasing the particle concentration around 10 wt%. See also the correspondingSupplementary Movie 3. Figure 5: Asymmetric Janus capsules after turning off the electric field. ( a , b ) Coalesced drops with equal material proportion. PE (50 μm green and red) particle concentration 7 wt% ( a ) and 10 wt% ( b ). The drops are non-spherical and remain so throughout the course of the experiment. ( c , d ) Coalesced drops with tuned material proportion. The original drops had different volumes (2:1 ratio) before coalescence. ( c ) Spherical capsule made of drops with 5 wt% particles, PE (green) and PS (white). ( d ) The bulb-like capsule was achieved by increasing the particle concentration around 10 wt%. See also the corresponding Supplementary Movie 3 . Full size image The shape of the arrested structure as well as the timing of the arresting process is determined by the particle surface coverage of the two original drops. The PE particle concentrations used for the merged drops in Fig. 5a,b are ~\n7 and 10% of the drop weight (hereafter denoted as wt%), resulting in ellipsoidal (a) and dumb-bell-like capsules (b), respectively. As shown in Supplementary Fig. 4 , these shapes remain stable also when the electric field is turned off. The proportion of materials on a shell may be tuned. This is shown in Fig. 5c,d , where PE and polystyrene (PS) particle-covered arrested shells were made from coalescing two drops, one with PE particles and the other with PS particles. The original drops had different original volumes (2:1 ratio) before electro-coalescence. The spherical capsule ( Fig. 5c ) was made from two original drops with 5 wt% particles and the non-spherical capsule ( Fig. 5d ) was made from two original drops with a 10 wt% particle concentration. Supplementary Movie 3 shows the arrested coalescence of the two droplets in Fig. 5d . We observe that micron- and sub-micron-sized particles can form stable non-spherical Janus capsules. In Fig. 6a the two hemispheres consist of glass (500 nm) and blue PE (20 μm) particles, whereas in Fig. 6b PS (1 μm) and clay colloidal minerals (~\n1 μm) particles are used. 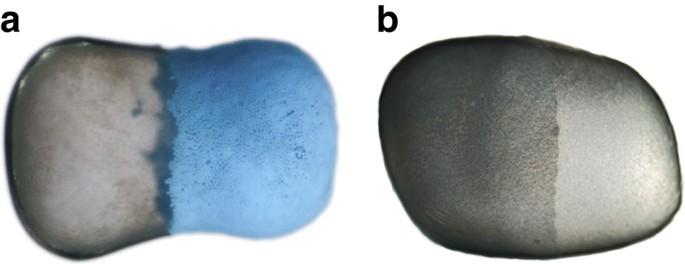Figure 6: Asymmetric Janus colloidal capsules. (a) Non-spherical Janus colloidal capsules with hemispheres consisting of glass (500 nm) and blue PE (20 μm) particles; (b) with PS (1 μm) and clay mineral (~\n1 μm) particles used. These colloidal capsules have asymmetric permeability and conductivity. Figure 6: Asymmetric Janus colloidal capsules. ( a ) Non-spherical Janus colloidal capsules with hemispheres consisting of glass (500 nm) and blue PE (20 μm) particles; ( b ) with PS (1 μm) and clay mineral (~\n1 μm) particles used. These colloidal capsules have asymmetric permeability and conductivity. Full size image Multi-patchy capsules In Fig. 7a we demonstrate how we can design a striped patchy capsule by coalescing three drops. We also demonstrate that a multilayer patchy capsule can be made by subsequent addition of material, that is, a series of coalescence of new drops with adequate concentrations of particles, resulting in a final capsule as presented in Fig. 7b . The ribbon-like areas can be formed by particles with different sizes and shapes, giving it additional functionality. 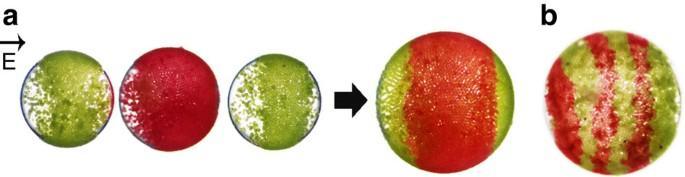Figure 7: Fabrication of patchy capsules. (a) Multilayer (three) shell made by coalescence of three drops. (b) Multilayer (six) striped patchy shell made by coalescence of six drops with adequate concentrations of PE particles. The size of the coalesced drops is ~\n2 mm. Figure 7: Fabrication of patchy capsules. ( a ) Multilayer (three) shell made by coalescence of three drops. ( b ) Multilayer (six) striped patchy shell made by coalescence of six drops with adequate concentrations of PE particles. The size of the coalesced drops is ~\n2 mm. Full size image Self-alignment of drops One final note on the assembly process is illustrated in Fig. 8 , which is that the drop coalescence is greatly aided by the spontaneous alignment and attraction of the drops dipoles in the DC electric field direction. This is in accordance with previous simulations [35] that suggest that drop dipole–dipole interactions dominate at short separation distances. EHD flow might also contribute to this alignment. 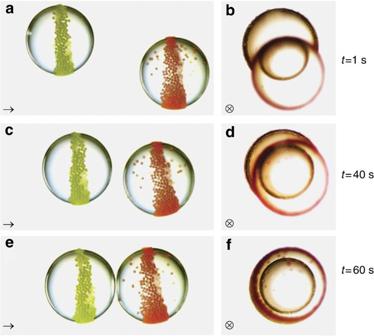Figure 8: Spontaneous alignment of drops before electro-coalescence. Drop coalescence is greatly aided by the self-alignment and attraction in the DC electric field along the polar axis, defined inFig. 1. The same two drops viewed perpendicular (a,c,e) and along (b,d,f) to the electric field direction are shown in the right and left panels, respectively. Arrows and crosses indicate the electric field direction, which coincide with induced dipole directions of the drops. In the right panels, the droplet covered with green particles appears smaller due to the optical lens effect looking through the droplet covered with red particles. The dipole–dipole interaction results in almost perfect alignment of the drops. Figure 8: Spontaneous alignment of drops before electro-coalescence. Drop coalescence is greatly aided by the self-alignment and attraction in the DC electric field along the polar axis, defined in Fig. 1 . The same two drops viewed perpendicular ( a , c , e ) and along ( b , d , f ) to the electric field direction are shown in the right and left panels, respectively. Arrows and crosses indicate the electric field direction, which coincide with induced dipole directions of the drops. In the right panels, the droplet covered with green particles appears smaller due to the optical lens effect looking through the droplet covered with red particles. The dipole–dipole interaction results in almost perfect alignment of the drops. Full size image In this paper we present and demonstrate a simple route for design of multi-patchy capsules, which is straightforward, robust and relies neither on direct electric forces acting on the colloidal particles nor on how the colloidal particles are brought to the droplet surfaces. It uses the simultaneous action of EHD flow and electro-coalescence. This assembly route serves as a starting point for producing colloidosomes with controlled patchiness, permeability and electric properties. Patchy colloidal shells can be sintered, as reported for homogenous colloidal shells [24] , [38] , eventually forming cohesive colloidal patchy shells. The EHD pre-structuring of particles into ordered ribbons is central in our method and ensures packed and sharply defined Janus and patchy capsules immediately after drop coalescence. Our method is distinctly different from previous work reported in the literature, where electro-coalescence has been used to merge drops containing different particles, which subsequently have been positioned by dielectrophoresis to make partly covered Janus drops rather than fully covered Janus capsules [39] . The capillary binding of a particle to a drop interface is proportional to the particle surface area, and therefore smaller particles might detach from the drop interface, that is, the chance of producing non-spherical Janus capsules is reduced when particle sizes go down to a few nanometres. It has been shown previously that non-spherical capsules can be produced with 100-nm-sized particles [37] , [40] . Our results can open new pathways towards formation of new architectures and structures, such as in controlling production of light and hollow scaffolds based on assemblies of colloidosomes with directed patchiness [41] . Electric field manipulation of droplets is often integrated in microfluidic circuits, and controlled mass production of patchy capsules can be achieved by using our electro formation method in conjunction with microfluidic droplet control [42] , [43] , [44] . Mass production in bulk might also be possible by mixing two populations of drops, and induce electro-coalescence, which can produce a mixture of Janus and homogenous shells. The Janus shells might subsequently be separated out based on differences, for example, in surface charge, dielectrophoretic or magnetic properties. We foresee that this route for designing patchy shells will facilitate foundation for many advanced applications, for example, by using previously reported microfluidic methods [45] . Finally, we note that our method also can be used to produce patchy particles, rather than patchy shells, by core solidification at the end of the route. Sample cell The experiments are performed in a square glass cuvette (10 × 10 × 30 mm), in which two sides are made of transparent ITO (indium tin oxide) electrodes, allowing observation of drops both parallel and perpendicular to the applied electric field. In all images, the direction of gravity is downward. The drops were placed in the middle of the sample cell. The sedimentation velocity of a drop was in all cases very small compared with the EHD velocities (see Supplementary Fig. 5 ). We also made drops comprising a mixture of 10 and 100 cSt silicone oils to density match the silicone drop with the castor oil. This resulted in sedimentation velocities ~\n0.001 mm s −1 . However, this did not change the dynamics of capsule formation. Standard stereomicroscopes Zeiss Stemi-2000C were used in all experiments. Oils The cell is filled with castor oil (Sigma-Aldrich 83912, specific density of 0.961 g cm −3 at 25 °C, electric conductivity 45 pS m −1 , relative permittivity 4.7 and viscosity 1,000 cSt). Silicone drops (Down Corning 200/100 cSt, Prod 630074A, specific density of 0.97 g cm −3 , electric conductivity ~\n3–5 pS m −1 , relative permittivity 2.1) containing particles are placed into the castor oil by using a pipette. Particles Fluorescent PE particles (UVPMS-BY2 45–53 μm) were purchased from Cospheric LLC; PS particles (Dynoseeds CS40) of diameter 40 μm were purchased from Microbeads. Fluorohectorite is a synthetic 2:1 clay mineral. The fluorohectorite clay mineral colloidal particles used here are polydisperse disk-shaped particles with average diameter ~\n1 μm, and average thickness of ~\n100 nm comes from the same batch of materials as reported and characterized previously by our group [46] . Silica microspheres with different diameters (0.5 and 1 μm) were purchased from Microspheres-Nanospheres. Preparation of dispersions Silicone oil and particles are measured by weight and stirred together, followed by ultrasonic bath to avoid aggregation. Particle assembly on the ‘electric equator’ The particles can be brought to the drop interface by any suitable method of choice. Once the particles are on the surface, electric-field-induced liquid flows (EHDs) assemble them rapidly into the ribbon located at the ‘electric equator’ of the drop. In Supplementary Fig. 5 we plot the average velocity ‹ v › of particles moving from the ‘electric poles’ to the ‘electric equator’ versus electric field strength squared, E 2 , as predicted in the Taylor–Melcher EHD model for leaky dielectric drops [28] . How to cite this article: Rozynek, Z. et al . Electroformation of Janus and patchy capsules. Nat. Commun. 5:3945 doi: 10.1038/ncomms4945 (2014).